Surface-redox sodium-ion storage in anatase titanium oxide Sodium-ion storage technologies are promising candidates for large-scale grid systems due to the abundance and low cost of sodium. However, compared to well-understood lithium-ion storage mechanisms, sodium-ion storage remains relatively unexplored. Herein, we systematically determine the sodium-ion storage properties of anatase titanium dioxide (TiO 2 (A)). During the initial sodiation process, a thin surface layer (~3 to 5 nm) of crystalline TiO 2 (A) becomes amorphous but still undergoes Ti 4+ /Ti 3+ redox reactions. A model explaining the role of the amorphous layer and the dependence of the specific capacity on the size of TiO 2 (A) nanoparticles is proposed. Amorphous nanoparticles of ~10 nm seem to be optimum in terms of achieving high specific capacity, on the order of 200 mAh g −1 , at high charge/discharge rates. Kinetic studies of TiO 2 (A) nanoparticles indicate that sodium-ion storage is due to a surface-redox mechanism that is not dependent on nanoparticle size in contrast to the lithiation of TiO 2 (A) which is a diffusion-limited intercalation process. The surface-redox properties of TiO 2 (A) result in excellent rate capability, cycling stability and low overpotentials. Moreover, tailoring the surface-redox mechanism enables thick electrodes of TiO 2 (A) to retain high rate properties, and represents a promising direction for high-power sodium-ion storage. Pseudocapacitive materials store charge through Faradaic reactions at rapid rates, offering a route for achieving both high energy and power densities [1] , [2] , [3] . In addition to well-known H + and Li + systems, pseudocapacitive materials can also reversibly store charge in “beyond-lithium” systems including Na + , K + , and Zn 2+ [4] , [5] , [6] , [7] , [8] , [9] , [10] . Pseudocapacitive storage is especially promising for high-rate sodium-ion storage which could enable technologies such as large-scale grid storage [11] , [12] , [13] , [14] . Pseudocapacitive mechanisms include surface-redox pseudocapacitance and intercalation pseudocapacitance [1] , [15] . Surface-redox pseudocapacitance occurs when Faradaic charge transfer processes take place at or near the surface of a material [3] , [4] . Intercalation pseudocapacitance is a bulk phenomenon, similar to battery-type intercalation. Both pseudocapacitive responses are characterized by capacitor-like electrochemical signatures and their kinetic behavior is not dominated by diffusion controlled processes [16] , [17] , [18] . Interestingly, certain intercalation materials for lithium-ion batteries demonstrate pseudocapacitive behavior when their particle size is reduced to several nanometers (termed extrinsic pseudocapacitive materials) [1] , [3] , [4] , [19] . One of these materials is anatase TiO 2 (TiO 2 (A)) [20] , [21] . TiO 2 (A) has a tetragonal crystal structure with empty octahedral sites that reversibly accommodate Li + intercalation and extraction [22] . Briefly, Li + intercalation into TiO 2 (A) occurs in three steps: solid solution (formation of α -Li x TiO 2 ), phase transformation from α -Li x TiO 2 to β -Li x TiO 2 (with a plateau at ~1.75 V vs . Li + /Li), and interfacial storage (from 1.7 to 1 V vs . Li + /Li) [21] . Research groups report that the specific capacity of TiO 2 (A) for lithium-ion storage is size-dependent arising from the slow Li + diffusion in the β -Li x TiO 2 [22] , [23] . In addition, when the particle sizes of TiO 2 (A) were reduced to ~7 nm, surface-controlled reactions due to the “nanosize effect” led to enhanced rate capability [20] . TiO 2 (A) also shows promising sodium-ion storage performance [24] , [25] , [26] , [27] , [28] , [29] , [30] , [31] , [32] , [33] , [34] , however, results regarding the sodium-ion storage mechanism of TiO 2 (A) are inconsistent. Previous literature showed that ex-situ [24] , [25] and in-situ [29] X-ray diffraction (XRD) patterns display unchanged diffraction peaks of crystalline TiO 2 (A) in both sodiated and desodiated states. In contrast, other publications based on the observation of small sized TiO 2 (A) nanoparticles (NPs), have indicated a complete loss of crystallinity after initial sodiation to 0.01 V vs . Na + /Na with the amorphous state maintained during subsequent cycles [30] . These two different responses lead to two conflicting explanations: the former proposed an intercalation mechanism without phase changes [24] , [25] , [29] , while the latter indicated an irreversible transition from crystalline TiO 2 (A) into an amorphous phase after the initial sodiation [30] . Although previous results showed different specific capacities of various TiO 2 (A) nanomaterials [24] , [25] , [26] , [27] , [28] , [29] , [30] , [31] , [32] , [33] , [34] , the above two explanations do not give rise to a consistent model which details the relationships among the capacities, particle sizes, and charge storage mechanism. Additionally, the sodium-ion storage of TiO 2 (A) anodes were considered to have pseudocapacitive responses [30] , but it was not determined whether the pseudocapacitive response is extrinsic (caused by “nanosize effect”) or intrinsic (inherent capacitor-like charge kinetics) [1] , [3] . If we are to understand the sodium-ion storage mechanism for TiO 2 (A), the above results must be reconciled and a consistent model needs to be proposed. In this work, we systematically investigate the electrochemical properties of TiO 2 (A) with particle sizes ranging from 5 to 100 nm to better understand the sodium-ion storage mechanism. A combination of methods including ex-situ/in-situ XRD, ex-situ transmission electron microscopy (TEM), and ex-situ X-ray photoelectron spectroscopy (XPS) were used to characterize different-sized TiO 2 (A) nanoparticles (NPs). These results demonstrate that only a thin surface layer (~3 to 5 nm) of crystalline TiO 2 (A) NPs becomes amorphous upon the initial sodiation process and remains amorphous in subsequent cycles. Based on our finding, a surface-dependent charge storage model is proposed, that details the relationship between particle size and specific capacity, and reconciles the inconsistencies in the literature reported for bulk and nanomaterials. When the particle size is significantly larger than the amorphous surface layer, the XRD patterns remain unchanged [24] , [25] , while the XRD patterns show the disappearance of peaks when the particle size is less than 10 nm [30] . The kinetic analysis based on cyclic voltammetry (CV) measurements indicate an intrinsic surface-redox reaction mechanism, which is size-independent and exhibits capacitor-like kinetics. Electrochemically, we demonstrate high-rate capability and excellent cycling stability when TiO 2 is used as a pseudocapacitive, sodium-ion storage anode. Characterization of TiO 2 (A) NPs XRD patterns of the different-sized TiO 2 NPs are shown in Supplementary Fig. 1a . All diffraction peaks correlate to the anatase phase without any impurities. The average crystallite sizes of the TiO 2 -NPs were calculated according to the Scherrer formula [20] . 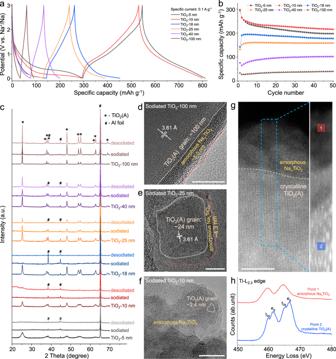Fig. 1: Structure and charge storage properties of various TiO2(A) NPs. The initial sodiation and desodiation curves (a) and cycling performance at 0.1 A g−1(b) of different TiO2NPs, respectively.cEx-situ XRD patterns of different TiO2NPs. Below 18 nm the (de)sodiated NPs are X-ray amorphous, whereas larger ones (>18 nm) remain crystalline. The ex-situ HRTEM images of TiO2-100 nm (d), TiO2−25 nm (e), and TiO2−10 nm (f) at the fully sodiated state, showing the amorphous NaxTiO2shell and crystalline TiO2(A) core structure. Scale bar: 10 nm. HAADF-STEM image (g) and EELS spectra of Ti-L2,3(h) of sodiated TiO2−25 nm. Scale bar: 5 nm. The calculated crystallite sizes of TiO 2 NPs and the corresponding Brunauer-Emmett-Teller (BET) surface areas of different TiO 2 are listed in Supplementary Table 1 . Assuming the NPs are spherical, the relationship between theoretical surface area ( S ) and particle sizes ( d ) follows S = dρ /6 [20] , where the density ( ρ ) of TiO 2 (A) is 3.82 g cm −3 . These calculated results (Supplementary Table 1 ) are consistent with the particle size observed by TEM (Supplementary Fig. 2 ). Influence of particle size on sodium-ion storage of TiO 2 (A) The electrochemical performance of different TiO 2 NPs is obtained using half cells with sodium metal as a counter/reference electrode. An electrolyte of 1 M NaPF 6 in diglyme was used as it promotes the formation of relatively thin SEI layers [30] , [31] . The specific capacity of TiO 2 NPs is carefully calculated to exclude the contribution from the conductive carbon additives (the detailed calculation steps are described in “Methods” section). Figure 1a shows the initial sodiation and desodiation curves of the six TiO 2 NPs at the specific current of 0.1 A g −1 (corresponding to the current density of 0.15 mA cm −2 ) in the potential window of 0.01–3 V vs. Na + /Na. The first cycle sodiation/desodiation capacities for the various NPs are listed in Table 1 . The specific capacity of TiO 2 -NPs is size-dependent with smaller sizes exhibiting higher capacity. Fig. 1: Structure and charge storage properties of various TiO 2 (A) NPs. The initial sodiation and desodiation curves ( a ) and cycling performance at 0.1 A g −1 ( b ) of different TiO 2 NPs, respectively. c Ex-situ XRD patterns of different TiO 2 NPs. Below 18 nm the (de)sodiated NPs are X-ray amorphous, whereas larger ones (>18 nm) remain crystalline. The ex-situ HRTEM images of TiO 2 -100 nm ( d ), TiO 2 −25 nm ( e ), and TiO 2 −10 nm ( f ) at the fully sodiated state, showing the amorphous Na x TiO 2 shell and crystalline TiO 2 (A) core structure. Scale bar: 10 nm. HAADF-STEM image ( g ) and EELS spectra of Ti-L 2,3 ( h ) of sodiated TiO 2 −25 nm. Scale bar: 5 nm. Full size image Table 1 The specific surface area and sodium-ion storage performance of different TiO 2 NPs at 0.1 A g −1 (0.15 mA cm −2 ) Full size table The cycling performance and the corresponding discharge-charge curves of the TiO 2 NPs at 0.1 A g −1 (0.15 mA cm −2 ) are shown in Fig. 1b and Supplementary Fig. S3 . TiO 2 -5 nm and TiO 2 -10 nm deliver a reversible specific capacity of ~265 mAh g −1 , corresponding to Na x TiO 2 ( x ≈ 0.8). Both materials show capacity fading during the initial cycles, but after ~10 cycles it is evident that TiO 2 -10 nm exhibits superior cycling stability compared with that of TiO 2 -5 nm. In contrast, the TiO 2 -18, 25, 40, and 100 nm anodes show an increase in specific capacity with repeated cycling. Ex-situ XRD patterns of different-size TiO 2 NPs are used to characterize the structural features during sodiation and desodiation (Fig. 1c ). A complete lack of crystallinity was observed for sodiated and desodiated TiO 2 -5, 10, and 18 nm (the peaks at 38.5°, 44.7° and 65.2° are from Al foil current collector), while the diffraction peaks are broadened but unchanged for the sodiated and desodiated TiO 2 −25, 40, and 100 nm. The loss of crystalline structure is not recovered in the subsequent desodiation process. Ex-situ high-resolution TEM (HRTEM) was used to further investigate the amorphous transitions. The sodiated TiO 2 -100 nm (Fig. 1d ) and TiO 2 -25 nm (Fig. 1e ) display the amorphous Na x TiO 2 shell and crystalline TiO 2 (A) core structure with a shell thickness of ~5.0 and 4.3 nm, respectively. In comparison, the HRTEM image of sodiated TiO 2 -10 nm (Fig. 1f ) displays a lack of long-range order with ultrafine TiO 2 (A) grains (~2 nm). Additionally, high-angle annular dark-field scanning transmission electron microscopy (HAADF-STEM) image of the sodiated TiO 2 -25 nm (Fig. 1g ) confirms the amorphous surface layer and crystalline core. Electron energy loss spectroscopy (EELS) spectra of Ti-L 2,3 edges (Fig. 1h ) show that the crystalline core (point 2 in Fig. 1g ) remains with the typical peaks of anatase TiO 2 , while, the peaks from surface amorphous Na x TiO 2 (point 1 in Fig. 1g ) indicate the reduction of surface Ti 4+ after sodiation [35] , [36] . It should be noted that acid treatment has been used to remove SEI layers [37] , [38] . This treatment does not influence the phase and surface structure of TiO 2 (A) NPs (Supplementary Fig. 4 ), and after acid treatment, the surface amorphous layers are also observed (Supplementary Fig. 5 ). These ex-situ HRTEM results indicate that the amorphous layers are from the electrochemical sodiation process, consistent with the loss of crystallinity observed by ex-situ XRD (Fig. 1c ). In-situ XRD was collected for two samples, TiO 2 -10 nm and TiO 2 -100 nm, to assess the structural changes associated with sodiation and desodiation. 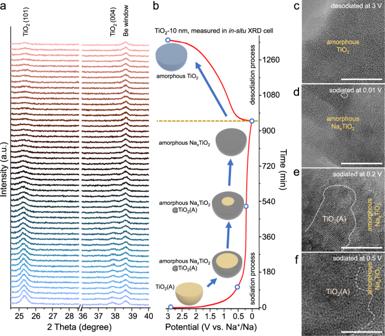Fig. 2: Structure evolution of TiO2-10 nm upon sodiation and desodiation. In-situ XRD patterns (a) and corresponding initial sodiation and desodiation curves at 0.03 A g−1(b) of TiO2-10 nm.cEx-situ HRTEM images of TiO2-10 nm desodiated at 3 V (c), and sodiated at 0.01 V (d), 0.2 V (e), and 0.5 V (f). The images indicate a continuous crystalline to amorphous transition at the particle surface which progresses inwards. Scale bar: 10 nm. Figure 2a shows the in-situ XRD patterns of TiO 2 -10 nm and the corresponding initial sodiation and desodiation curves (Fig. 2b ) at 0.03 A g −1 (0.045 mA cm −2 ). The first sodiation curve of the TiO 2 -10 nm anode displays a plateau at ~0.25 V vs . Na + /Na. At this potential, the TiO 2 (101) and (004) peaks do not shift upon initial sodiation, but broaden and disappear with additional sodiation. This series of XRD scans indicates that the TiO 2 transitions from a crystalline to an amorphous state upon the sodiation plateau. In the subsequent desodiation process, the TiO 2 remains in the amorphous state, and the galvanostatic charge profile displays a curved slope, which is typical of pseudocapacitive charge storage behavior [1] , [3] . Additionally, ex-situ HRTEM images of TiO 2 -10 nm at different sodiation states (Fig. 2c–f ) indicate a continuous crystalline to amorphous transition at the particle surface which progresses inward (schematically shown in Fig. 2b ). Fig. 2: Structure evolution of TiO 2 -10 nm upon sodiation and desodiation. In-situ XRD patterns ( a ) and corresponding initial sodiation and desodiation curves at 0.03 A g −1 ( b ) of TiO 2 -10 nm. c Ex-situ HRTEM images of TiO 2 -10 nm desodiated at 3 V ( c ), and sodiated at 0.01 V ( d ), 0.2 V ( e ), and 0.5 V ( f ). The images indicate a continuous crystalline to amorphous transition at the particle surface which progresses inwards. Scale bar: 10 nm. Full size image In contrast, the TiO 2 -100 nm shows a rather limited sodiation characteristic, with no evidence of a plateau and with a curved galvanostatic discharge-charge profile (Fig. 1a and Supplementary Fig. 3f ). Moreover, the in-situ XRD patterns exhibit no change in the crystalline phase of anatase during six cycles (Supplementary Fig. 6 ). The two different results for TiO 2 -10 nm and TiO 2 -100 nm indicate that the particle sizes have a significant influence on the electrochemical sodium-ion storage which may explain the discrepancies of XRD peaks in previously reported data [24] , [25] , [29] , [30] . This finding is consistent with the ex-situ XRD patterns of different-size TiO 2 NPs (Fig. 1c ). Ex-situ Ti 2p XPS spectra of TiO 2 -10 nm and TiO 2 -100 nm (Supplementary Figs. 7 , 8 and Supplementary Table 2 ) show the reversible redox of Ti 4+ /Ti 3+ during sodiation and desodiation. It is significant to note that both materials exhibit the presence of the similar amorphous surface composition (Na x TiO 2 with x = 0.8). Moreover, neither metallic Ti nor Na 2 O were observed in the ex-situ XPS spectrum, ex-situ XRD, or TEM results. This is consistent with the findings of Siebert et al. [39] who demonstrated the reversible Ti 4+ /Ti 3+ redox reaction through operando X-ray absorption near-edge structure spectroscopy (XANES) of the Ti K-edge. Additionally, extended X-ray absorption fine structure (EXAFS) indicated the coexistence of Ti 4+ –O and Ti 3+ –O bonds after sodiation and the reversible shrinkage of Ti–O bonds after desodiation [30] . These results confirm that the sodium-ion storage of TiO 2 (A) is not a conversion reaction and is exclusively based on the Ti 4+ /Ti 3+ redox couple. The sodium-ion storage mechanism of TiO 2 (A) is summarized schematically in Fig. 3a . The initial sodiation of TiO 2 (A) involves a gradual surface amorphization process, but importantly, the reaction depth is only ~3 to 5 nm. The surface-sodiated compositions of different-sized NPs are consistent, Na 0.80 TiO 2 . After the initial sodiation, the following charge/discharge cycles rely on the redox properties of the surface Na x TiO 2 . This mechanism explains the different observations for in-situ/ex-situ XRD patterns (Fig. 1c , Fig. 2a and Supplementary Fig. 6 ) and previous reports [24] , [25] , [29] , [30] . Since the amorphization is on the order of ~3 to 5 nm, the TiO 2 -10 nm completely transforms into an amorphous material leading to the disappearance of XRD peaks (Figs. 1c and 2a ) and the long initial sodiation plateau (Fig. 1a ). The particle cores of the TiO 2 NPs over 25 nm, however, remain largely intact, resulting in well-defined XRD peaks throughout cycling (Fig. 1c ). Fig. 3: Overview of the sodium-ion storage mechanism of TiO 2 (A). a For particles >10 nm, only a thin surface layer of crystalline TiO 2 (A) is amorphized at the initial sodiation process, producing the sodiated amorphous composition of Na x TiO 2 ( x = 0.80). For particles <10 nm, they totally tend into amorphous state. The materials remain in the amorphous state with reversible redox of Ti 4+ /Ti 3+ in the following cycles. b, c A model fitting the particle size, delivered specific capacity and reaction thickness of the TiO 2 NPs. The sodiated surface layer produces a high capacity ( Q 0 = 265 mAh g −1 ), but the specific capacity of the entire TiO 2 particle depends on the proportion of the reaction thickness ( h ) to the total spherical diameter ( D ). The measured reversible specific capacity of different-sized TiO 2 (this work and refs. 27 , 30 , 32 , 33 , 34 ) fit well with the reaction thickness of 3–5 nm, which is consistent with the experimental observations. The limited surface reaction thickness is responsible for the particle size dependence of the specific capacity. Full size image Because of the limited surface-reaction thickness, the specific capacity is largely dependent on particle size. TiO 2 NPs deliver maximum capacity when the particle size is below 10 nm and the specific capacity decreases rapidly when the NP size is increased. Here, a mathematic model is proposed (Fig. 3b ) based on a core-shell structure of the spherical particle. Assuming the reacted surface shell delivers the same capacity ( Q 0 ) for each material, the specific capacity of a given TiO 2 particle is dependent on the proportion of the reaction thickness ( h ) to the total spherical diameter ( D ). 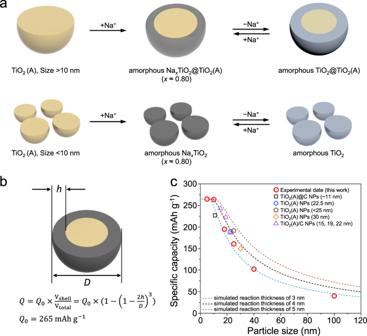Fig. 3: Overview of the sodium-ion storage mechanism of TiO2(A). aFor particles >10 nm, only a thin surface layer of crystalline TiO2(A) is amorphized at the initial sodiation process, producing the sodiated amorphous composition of NaxTiO2(x= 0.80). For particles <10 nm, they totally tend into amorphous state. The materials remain in the amorphous state with reversible redox of Ti4+/Ti3+in the following cycles.b, cA model fitting the particle size, delivered specific capacity and reaction thickness of the TiO2NPs. The sodiated surface layer produces a high capacity (Q0= 265 mAh g−1), but the specific capacity of the entire TiO2particle depends on the proportion of the reaction thickness (h) to the total spherical diameter (D). The measured reversible specific capacity of different-sized TiO2(this work and refs.27,30,32,33,34) fit well with the reaction thickness of 3–5 nm, which is consistent with the experimental observations. The limited surface reaction thickness is responsible for the particle size dependence of the specific capacity. Figure 3c shows the simulated curves based on the relations among the reaction thickness ( h ), particle size ( D ), and the obtained specific capacity ( Q ). The measured reversible specific capacity (Supplementary Table 3 ) for different TiO 2 NPs, previously reported TiO 2 (A) nanoparticles [27] , [30] , [32] , [33] and olive-shaped TiO 2 (A) NPs/carbon composites (TOC) with various sizes (~15, 19 and 22 nm) [34] fit well for an assumed reaction thickness between 3 and 5 nm. This response is consistent with experimental observations (Fig. 1d–f ). Sodium-ion storage processes for TiO 2 To achieve better understanding of the sodium-ion storage process for the TiO 2 NPs, a comparison was made with that of lithium-ion storage for the same range of TiO 2 NPs. Results for the full range of TiO 2 NPs for sodium-ion storage are presented in Supplementary Section 3 , Figs. 9 – 15 , while the corresponding TiO 2 NPs for lithium-ion storage are displayed in Supplementary Section 4 , Figs. 16 – 19 . 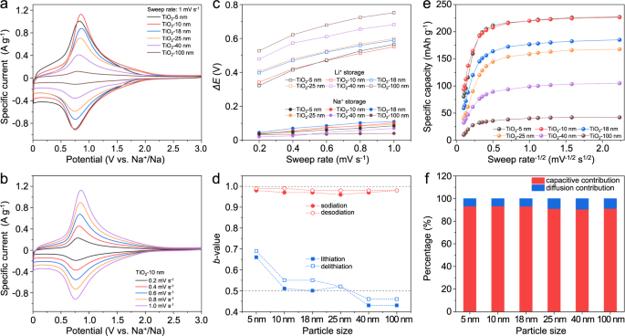Fig. 4: Charge storage properties of TiO2for lithium and sodium ions. aCV curves of the TiO2NPs at the sweep rate of 1.0 mV s−1showing small voltage offset between redox peaks.bCV curves of TiO2-10 nm at sweep rates of 0.2–1.0 mV s−1, indicating slight peak shifts with increasing sweep rates.cThe potential gap between the cathodic and anodic peaks (\(\varDelta E\)) as a function of particle size and sweep rate for Na+and Li+. A much smaller potential offset for sodium-ion storage is observed.dThe fittedb-values of the (de)sodiation and (de)lithiation peaks of TiO2NPs, where the\({b}_{{{{{{{\rm{Na}}}}}}}^{+}}\)≈1 indicates a capacitor-like process.eSpecific capacity vs.ν−1/2curves of the TiO2NPs.fThe capacitive and diffusion contributions for the TiO2NPs at the sweep rate of 1.0 mV s−1. Figure 4a shows that the CV curves for all TiO 2 NPs (at 1 mV s -1 ) exhibit similar redox peaks centered at ~0.75 V vs . Na + /Na, corresponding to the redox of Ti 4+ /Ti 3+ from the amorphous TiO 2 layer (as indicated by the ex-situ XPS, Supplementary Fig. 8 ). With the increase in sweep rates, the TiO 2 NPs show slight peak shifts (Fig. 4b and Supplementary Fig. 9 ). Even over narrow potential ranges, the TiO 2 anodes show the same redox peaks, indicating the highly reversible surface-redox reaction (Supplementary Fig. 10 ). The potential gap between the cathodic and anodic peaks ( \(\varDelta E\) ) for both sodium and lithium are shown as a function of particle size and sweep rate in Fig. 4c . At the sweep rate of 0.2 mV s −1 , the \({\varDelta E}_{{{{{{{\rm{Na}}}}}}}^{+}}\) of all NPs are <0.045 V, much smaller than those of \({\varDelta E}_{{{{{{{\rm{Li}}}}}}}^{+}}\) (>0.32 V). With the increase of sweep rates, the \({\varDelta E}_{{{{{{{\rm{Na}}}}}}}^{+}}\) (<0.11 V at 1 mV s −1 ) are much lower than that of \({\varDelta E}_{{{{{{{\rm{Li}}}}}}}^{+}}\) (>0.55 V at 1 mV s −1 ) as well. The smaller potential offsets are typical for pseudocapacitive charge storage processes and very different from those of battery-type intercalation materials [1] , [3] . Fig. 4: Charge storage properties of TiO 2 for lithium and sodium ions. a CV curves of the TiO 2 NPs at the sweep rate of 1.0 mV s −1 showing small voltage offset between redox peaks. b CV curves of TiO 2 -10 nm at sweep rates of 0.2–1.0 mV s −1 , indicating slight peak shifts with increasing sweep rates. c The potential gap between the cathodic and anodic peaks ( \(\varDelta E\) ) as a function of particle size and sweep rate for Na + and Li + . A much smaller potential offset for sodium-ion storage is observed. d The fitted b -values of the (de)sodiation and (de)lithiation peaks of TiO 2 NPs, where the \({b}_{{{{{{{\rm{Na}}}}}}}^{+}}\) ≈1 indicates a capacitor-like process. e Specific capacity vs. ν −1/2 curves of the TiO 2 NPs. f The capacitive and diffusion contributions for the TiO 2 NPs at the sweep rate of 1.0 mV s −1 . Full size image The CV measurements were also used to characterize the kinetics of the charge storage process. In this analysis, the peak current \(({i}_{p})\) follows the power-law shown in Eq. 1 [19] : 
    i_p=aν^b
 (1) where the b -value of 0.5 refers to a semi-infinite diffusion process, and b = 1 indicates a surface-controlled or capacitor-like kinetics. The b -values for the sodium-ion and lithium-ion storage are calculated in Supplementary Figs. 11 and 17 , respectively. For lithium-ion storage of TiO 2 (A), the material is a well-known insertion-type anode and \({b}_{{{{{{{\rm{Li}}}}}}}^{+}}\) ≈ 0.5 (Fig. 4d ). When the TiO 2 -NP size is reduced into the nanometer range, the value of \({b}_{{{{{{{\rm{Li}}}}}}}^{+}}\) for TiO 2 -5 nm is increased to 0.69, consistent with previous reports [20] . In contrast, the \({b}_{{{{{{{\rm{Na}}}}}}}^{+}}\) values of all the TiO 2 NPs are very close to 1, signifying surface-controlled kinetics (Fig. 4d ). To further explore the nature of diffusion-controlled and capacitive charge storage behaviors, the Trasatti analysis (Eq. 2 ) method was used [13] . Q(υ)=Q_capacitive+α (υ^-1/2)
 (2) where α is a constant, and \(Q(\upsilon )\) refers to the measured capacity, \({Q}_{{{{{{\rm{capacitive}}}}}}}\) is capacitive charge storage, and \(\,{Q}_{{{{{{\rm{total}}}}}}}\) is the total amount of charge storage. For the sodium-ion storage of TiO 2 NPs, the capacity is relatively independent at sweep rates below 4 mV s −1 (Fig. 4e ), suggesting a capacitive type of process. In contrast, the capacities measured for lithium-ion storage tend to show a linear dependence on ν −1/2 which is consistent with a diffusion-controlled mechanism (Supplementary Fig. 18b ). A qualitative indication of the charge storage process can be obtained by separating the current response ( i ) into two contributions, namely capacitive ( k 1 ν ) and diffusion-controlled ( k 2 ν 1/2 ) (Eq. 3 ) [1] . i(υ)=k_1υ+k_2υ^1/2
 (3) Supplementary Fig. 12 shows that the current arises almost exclusively from a capacitive contribution for all TiO 2 NPs, at the sweep rate of 1 mV s −1 . That is, the total capacity is dominated by capacitive contributions (over 90%, Fig. 4f ). In a confirming experiment, a TiO 2 −10 nm thin-film electrode (100 μg cm −2 ) was prepared without any conductive carbon additive or binders [16] . In this way, the influence of these other additives was eliminated. The CV curves for this thin-film electrode (Supplementary Fig. 13 ) and the corresponding b > 0.9 from Eq. 1 show the same charge storage behavior as the electrodes containing binder and conductive additive. In addition, the electrochemical behaviors of different TiO 2 NPs measured in ester-based electrolyte (Supplementary Fig. 14 ) are consistent with the results of ether-based electrolyte. These results support the contention that the sodium-ion charge storage process for TiO 2 NPs is the intrinsic surface-redox mechanism that arises from the electrochemically formed amorphous surface layer, and is independent of the electrolyte system used in the experiments. The rate capabilities for sodium-ion storage for the various TiO 2 NPs are shown in Fig. 5a . The TiO 2 −10 nm material, in particular, shows good specific capacity at high-rates, with values of nearly 200 mAh g −1 at 1 A g −1 (1.5 mA cm −2 ). Even at 4 A g −1 (6 mA cm −2 ) the material stores nearly 160 mAh g −1 . The galvanostatic charge-discharge curves show little change in their profiles with increasing current density (Fig. 5b ). Moreover, the TiO 2 -10 nm anode exhibits excellent fast‑charging and high‑rate performance when it is measured under fixed charging or discharging rates (Supplementary Fig. 15 ). The TiO 2 -10 nm also shows stable long-term cycling performance (Fig. 5c ): the capacity retention is 90.0% after 5000 cycles at a specific current of 2 A g −1 (3.0 mA cm −2 ). During long-term cycling, the charge-discharge curves overlap well (Fig. 5d ) without an increase in overpotential, indicating sodium-ion storage in TiO 2 is highly reversible and stable. Fig. 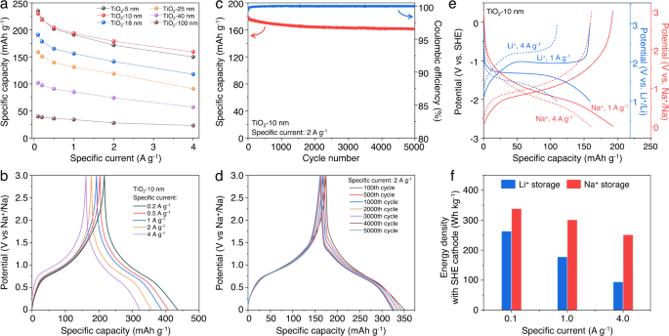Fig. 5: Sodium-ion storage properties of TiO2NPs. aRate capability of the different TiO2NPs.bCharge-discharge curves of the TiO2-10 nm at different specific currents, from 0.2 to 4 A g−1. Extended cycling (c) and related charge-discharge curves at various cycles (d) for the TiO2-10 nm at 2 A g−1. Excellent stability for 5000 cycles is shown.eThe charge and discharge curves of the TiO2-10 nm for Li+and Na+storagevs. SHE.fThe calculated average energy density for Li+and Na+storage for 10 nm TiO2NPs. The calculation is based on using SHE as a hypothetical cathode. The higher energy density for Na+storage at high power is very appealing for device applications. 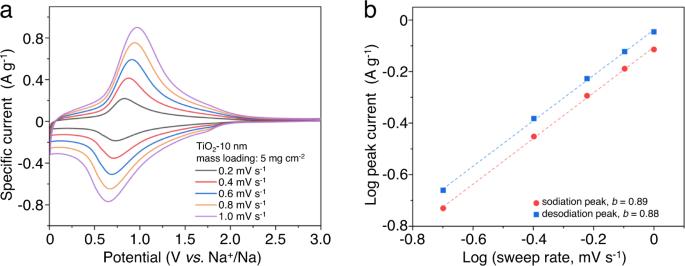Fig. 6: High-mass loading performance of TiO2NPs. The small voltage offset in CV curves (a) and theb-value analysis (b) of the TiO2-10 nm for 5 mg cm−2mass loading. The results indicate that surface-controlled kinetics also occur in thick electrodes. 5: Sodium-ion storage properties of TiO 2 NPs. a Rate capability of the different TiO 2 NPs. b Charge-discharge curves of the TiO 2 -10 nm at different specific currents, from 0.2 to 4 A g −1 . Extended cycling ( c ) and related charge-discharge curves at various cycles ( d ) for the TiO 2 -10 nm at 2 A g −1 . Excellent stability for 5000 cycles is shown. e The charge and discharge curves of the TiO 2 -10 nm for Li + and Na + storage vs . SHE. f The calculated average energy density for Li + and Na + storage for 10 nm TiO 2 NPs. The calculation is based on using SHE as a hypothetical cathode. The higher energy density for Na + storage at high power is very appealing for device applications. Full size image An anode material with high specific capacity and a low operating potential is beneficial to obtaining high energy density in a full cell. The operating potential of TiO 2 for sodium-ion storage (~0.75 V vs . Na + /Na, that is −1.96 V vs. standard hydrogen electrode (SHE)) is much lower than that of lithium-ion storage (~1.75 V vs. Li + /Li, that is −1.29 V vs. SHE) (Fig. 5e ). To numerically compare the energy density of the TiO 2 for both lithium-ion and sodium-ion storage, we calculated the energy density by using the SHE as a cathode reference, according to the methods suggested by Cao et al. [40] . By this methodology, the energy densities of TiO 2 -10 nm for sodium-ion storage (300 Wh kg −1 ) are higher than that of lithium-ion storage (176 Wh kg −1 ) (Fig. 5f ), at the high specific current of 1 A g −1 (1.5 mA cm −2 ). Moreover, at a higher specific current (4 A g −1 , 6.0 mA cm −2 ), the energy density of the TiO 2 -10 nm for sodium-ion storage exhibits much higher values than that for lithium-ion storage (250 vs . 93 Wh kg −1 ). Thick-film electrodes of TiO 2 -10 nm at a mass loading of 5 mg cm -2 were prepared in order to determine whether the greater mass would influence charge storage processes [41] . This thick electrode displays a similar CV response at varying sweep rates to those of 1.5 mg cm −2 (compare Fig. 6a with Fig. 4b ). At this high-mass loading level, the b -values (Fig. 6b ) determined from peak cathodic/anodic currents were on the order of 0.9, once again indicating surface-controlled kinetics. Taken together, these results for high mass loadings exhibit several pseudocapacitive signatures and offer the prospect of achieving high energy and high power, appealing features for practical applications. Fig. 6: High-mass loading performance of TiO 2 NPs. The small voltage offset in CV curves ( a ) and the b -value analysis ( b ) of the TiO 2 -10 nm for 5 mg cm −2 mass loading. The results indicate that surface-controlled kinetics also occur in thick electrodes. Full size image A combination of in-situ and ex-situ characterization has been used to determine the sodium-ion storage mechanism of TiO 2 (A) nanoparticles which range in size from 5 to 100 nm. The sodium-ion storage properties are attributed to the presence of surface layers of 3–5 nm thick. During the initial sodiation process, the surface layers of TiO 2 (A) become amorphous and subsequent Ti 4+ /Ti 3+ redox reactions in the amorphous titanium oxide surface layer lead to significant levels of charge storage. A model detailing the relationship between particle size and specific capacity is able to reconcile prior results in the literature which showed a very strong dependence on particle size. The best electrochemical performance occurs with small particles whose size (~10 nm) is such that nearly the entire particle is amorphous. These particles are X-ray amorphous whereas larger ones (>10 nm) remain crystalline. Kinetic studies exhibit several pseudocapacitive signatures as redox reactions occur at the surface and near surface regions. These properties include peak currents with linear dependence on sweep rate, charge storage which is relatively independent of sweep rate and a small voltage offset between oxidation and reduction reactions. The kinetics for sodium-ion storage in TiO 2 (A) are very different from those of lithium-ion processes as the surface-redox mechanism for sodium-ion storage is not limited by semi-infinite diffusion and exhibits excellent rate capability, cycle stability and low overpotentials. We find that the surface-redox mechanism is also active in thick electrodes, which is promising for practical applications. TiO 2 nanoparticles The TiO 2 (anatase) nanoparticles are purchased from US Research Nanomaterials, Inc., and used without additional treatment. Material characterizations The powder X-ray diffraction (XRD) was characterized on Bruker-Axs X-ray diffractometer (Cu Kα radiation, λ = 1.5406 Å). In-situ XRD was measured by using a customized two-electrode cell, in which a piece of Be disk were used as the current collector and the X-ray transparent window. Brunauer-Emmet-Teller (BET) specific surface area was measured by nitrogen sorption isotherms (Micromeritics Tristar 3020) at 77 K after degassed under vacuum at 200 °C for over 6 h. Transmission electron microscopy (TEM) images were recorded by using Titan G2 60–300. The high-angle annular dark-field scanning transmission electron microscopy (HAADF-STEM) images and electron energy loss spectroscopy (EELS) spectra were obtained through double spherical aberration corrected transmission electron microscope (Titan Cubed Themis G2 300). For the powder samples, the TiO 2 NPs were sonicated in alcohol and dropped onto the grid for TEM observation. For preparing the ex-situ TEM samples, the coin cells were disassembled in an Ar-filled glove box after being electrochemically cycled at different states, and the electrodes were washed with the diglyme solvent. Then, the TiO 2 NPs were carefully scratched from the Al foil, sonicated in diglyme and dropped onto the grid for TEM observation. For preparing the ex-situ TEM sample with removed SEI layers, the electrodes were washed with the diglyme solvent. Then, the TiO 2 NPs were carefully scratched from the Al foil and soaked in 0.1 M HCl solution for 1 h. After centrifuging, the washed sample was sonicated in alcohol and dropped onto the grid for TEM observation. XPS survey scan analyses were conducted on a Kratos Axis Supra using monochromatized Al Kα X-ray source (1486.7 eV). The XPS chamber was directly connected to the Ar-filled grove box to avoid air exposure during sample preparation and transfer. The coin cell was disassembled in the Ar-filled glove box after electrochemically cycled at different states, and the TiO 2 NPs electrode was washed with the diglyme solvent. After drying, the anodes were transferred to the XPS chamber for testing. Spectra were charge corrected to the main line of the carbon 1 s spectrum and set to a binding energy of 284.8 eV. Electrode preparation and electrochemical measurement The TiO 2 electrodes were made from an aqueous slurry consisting of 85 wt.% TiO 2 NPs, 7 wt.% Ketjen black, 4 wt.% carboxyl methyl cellulose (CMC) and 4 wt.% styrene butadiene rubber (SBR). For sodium-ion storage measurements, the slurry was cast onto Al foil using doctor blading. For lithium-ion storage measurements, the slurry was cast onto Cu foil. The coated slurry was dried at 120 °C under vacuum for 12 h. The mass loading of different-sized TiO 2 electrodes were controlled at ≈1.5 mg cm −2 . To measure the electrochemical performance of TiO 2 -10 nm at very thick films, the loading was increased to 5 mg cm −2 . Coin cells (CR2032) were assembled in an Ar-filled glove box. For sodium-ion storage measurements, the sodium metal disk was used as the counter and reference electrode, Celgard-2325 used as separator, and 1 M NaPF 6 in diglyme used as electrolyte. For lithium-ion storage measurements, lithium metal disk was used as counter and reference electrode, Celgard-2325 as separator, 1 M LiPF 6 in ethylene carbonate (EC)/dimethyl carbonate (DMC) with a volume ratio of 50:50 as the electrolyte. Electrochemical measurements were carried out by Bio-Logic VSP potentiostat. For sodium-ion storage, the potential window is set in 0.01–3 V vs . Na + /Na. For lithium-ion storage, the potential window is set in 1–3 V vs . Li + /Li. All the coin cells were placed in an incubator with a stationary temperature of 25 °C for electrochemical measurements. Calculation the specific capacity of TiO 2 NPs The composite electrodes consist of 85 wt.% TiO 2 NPs, 7 wt.% carbon additive (Ketjen black) and 8 wt.% binders (CMC + SBR). The total capacity of electrode \({Q}_{{{{{{\rm{total}}}}}}}={Q}_{{{{{{{\rm{TiO}}}}}}}_{2}}+{Q}_{{{{{{\rm{carbon}}}}}}}={Q}_{{{{{\rm{S}}}}},{{{{{{\rm{TiO}}}}}}}_{2}}\times {m}_{{{{{{{\rm{TiO}}}}}}}_{2}}+{Q}_{{{{{\rm{S}}}}},{{{{{\rm{carbon}}}}}}}\times {m}_{{{{{{\rm{carbon}}}}}}}\) . As a rigorous approach to isolate the capacity from the TiO 2 alone, additional sodiation capacity from the conductive carbon additive is measured for removal. The reversible specific capacity of carbon additive ( \({Q}_{{{{{{\rm{S}}}}}},{{{{{\rm{carbon}}}}}}}\) ) is 124 mAh g −1 at 0.05 A g −1 in the potential range of 0.01–3 V vs. Na + /Na, through making an electrode only consisting of carbon additives and binders. Then, by removing the contribution from the carbon additives, the specific capacity of TiO 2 ( \({Q}_{{{{{{\rm{S}}}}}},{{{{{{\rm{TiO}}}}}}}_{2}}\) ) is calculated according to the following Eqs. 4 and 5 . Q_S,TiO_2=(Q_total-124mAhg^-1×m_carbon)/m_TiO_2
 (4) 
    Q_S,TiO_2=(Q_total-124mAhg^-1×0.07m_total)/0.85m_total
 (5) Calculation the energy density of TiO 2 versus SHE reference The energy densities ( E ) of TiO 2 anodes for both lithium-ion and sodium-ion storages were calculated by using the standard hydrogen electrode (SHE) as the hypothetical cathode [40] . The galvanostatic desodiation (or delithiation) curves were applied for integrating based on \(E=\int {{{{{\rm{I}}}}}}{{{{{\rm{V}}}}}}{dt}\) , while the potential (V) versus SHE was applied.